Customized reaction route for ruthenium oxide towards stabilized water oxidation in high-performance PEM electrolyzers The poor stability of Ru-based acidic oxygen evolution (OER) electrocatalysts has greatly hampered their application in polymer electrolyte membrane electrolyzers (PEMWEs). Traditional understanding of performance degradation centered on influence of bias fails in describing the stability trend, calling for deep dive into the essential origin of inactivation. Here we uncover the decisive role of reaction route (including catalytic mechanism and intermediates binding strength) on operational stability of Ru-based catalysts. Using MRuO x (M = Ce 4+ , Sn 4+ , Ru 4+ , Cr 4+ ) solid solution as structure model, we find the reaction route, thereby stability, can be customized by controlling the Ru charge. The screened SnRuO x thus exhibits orders of magnitude lifespan extension. A scalable PEMWE single cell using SnRuO x anode conveys an ever-smallest degradation rate of 53 μV h −1 during a 1300 h operation at 1 A cm −2 . Water electrolysis using a polymer electrolyte membrane (PEM) is deemed most suitable to propel a carbon-neutral future by converting the intermittent renewable energy resources into high purity H 2 [1] , [2] , [3] , [4] , [5] , due to its innate advantages over alkaline water electrolyzer in terms of current density and instant current response [6] , [7] , [8] . In practice, however, large-scale deployment of PEM water splitting is greatly constrained by the water oxidation catalysis half-reaction, which provides protons and electrons for hydrogen production [9] , [10] , with two essential limitations: (i) the high capital cost of scarce and expensive Ir (US$60,670 kg −1 ) catalysts currently used [11] , [12] ; (ii) the high overpotentials and thereby low energy efficiency of Ir in catalyzing the oxygen evolution reaction (OER) [13] . These two limitations in combination make Ir-based catalysts difficult to meet the 2025 goal of the US Department of Energy (DOE) (H 2 production cost <US $2 kg H2 −1 ) [14] , [15] . Given this, Ru has attracted research interests worldwide with lower prices (US$9,523 kg −1 ), higher earth abundance, and higher intrinsic OER activity [16] , [17] , [18] . However, the inferior dissolution resistance of Ru oxides in harsh anodic and acidic conditions remains long-unsolved, making it unrealistic for practical utilization due to the limited lifespan of only dozens of hours [19] , [20] , [21] , [22] . Thus, improving the operational stability of Ru-based catalysts is highly desired [23] . The lack of pertinent descriptors that could successfully capture the essential origin of the Ru inactivation in operation conditions has led to slow progress in stability improvement [24] . Since 1966, the over-oxidation of Ru to volatile RuO 4 or soluble RuO 5 2− at a high potential (>1.4 V) has been claimed responsible for its poor stability according to the Pourbaix diagram [25] , [26] , [27] . Thereafter, two main strategies, i.e., either introducing electron-donating elements to lower the Ru oxidation state at fixed anodic potential [28] , [29] , [30] , [31] or enhancing the intrinsic activity to reduce the working potential of the catalysts, were adopted to extend operating life [21] , [32] . Such efforts, however, have led to only limited progress despite decades of study, and these ideas centered on the influence of bias have been challenged by a few observations in recent years. First, despite that some electron-donating elements (Sr, La, Mn, Ce, etc.) can increase the proportion of low-valent Ru species (i.e., Ru 3+ ) and effectively suppress the Ru over-oxidation, inferior operating stabilities were still achieved on these catalysts that bind oxygen too weakly [33] , [34] , [35] , [36] . Second, it was only recently, with technological advances allowing for precise reaction mechanism probing, that the involvement of lattice oxygen in OER [37] has been identified as one major cause for the extremely poor stability according to the previous work from Wohlfahrt-Mehrens and Heitbaum, in spite of boosted activity [18] , [38] , [39] , [40] , [41] . These demonstrations highlight the importance of the long-ignored role of the OER routes (including the reaction mechanism and binding strength of intermediates) in determining catalyst durability. However, delineating the path to constructing a well-stabilized catalyst is still highly challenging and obstructed, as it would require the development of a universal descriptor that could embody both the reaction path and binding energies in a sole structural parameter, which is currently unavailable [42] , [43] . Herein, we present an intuitive descriptor, i.e., the Ru charge, to describe the overall activity and stability of the catalysts. We reveal that, despite the complexity, catalyst destabilization is in close association with Ru charge and level of difficulty in Ru-O bond breaking, i.e., the balance of formation energy between oxygen vacancy (Δ G VO ) and the Ru vacancy (Δ G VRu ). By varying the chelating elements surrounding the RuO6 motif via controlling the M-O-Ru structure, we succeeded not only in regulating the reaction mechanism, i.e., choosing either or not to involve the lattice oxygen into the reaction (LOM, supplementary Fig. 1a ) [44] , [45] , but also in tailoring the activity and stability under adsorbate evolution reaction (AEM, supplementary Fig. 1b ) [46] . Guided by this understanding, we screened out SnRuO x solid solution with Sn-O-Ru local structure that follows the AEM with appropriate Ru-O binding strength. The SnRuO x catalysts exhibit the high intrinsic activity of 2360 A g Ru −1 at 1.48 V vs. RHE, with TOF representing the highest value reported for the catalysts following the AEM mechanism, i.e., 0.63 s −1 . Moreover, the catalyst exhibits the best operational stability to date, with only a 26.8 mV increase in overpotential during the 250 h test under 100 mA cm −2 at a low catalyst loading of 41.65 μg cat cm −2 . In a scalable PEM electrolyzer, an ever-smallest degradation rate of 53 μV h −1 is demonstrated during a 1300 h durability test at 1 A cm −2 , which successfully extends the lifespan of Ru-based catalysts by orders of magnitude, thus unambiguously validating our idea to improve the stability. We put forward a feasible idea to construct a stable and highly-efficient Ru-based OER catalyst, which laid the foundation for the application of Ru-based materials in PEMWE. Rational design of the intuitive descriptor We initiate by recognizing the lack of pertinent physical parameters to describe the overall performance of the Ru-based catalysts, irrespective of the reaction mechanism. Previously, reactivity descriptors, including the e g filling [47] , [48] , d band center [28] , p band center [11] , and the adsorption energy difference between catalytic sites and dopants proposed by ref. [49] . were found feasible in describing the activity trend of the catalysts following either the AEM or LOM mechanism. However, a unified scale, which comprises information on activity and stability in combined reaction mechanisms (both AEM and LOM), is lacking, thereby obscuring the advancing direction of the catalysts. We reasoned that, despite the complexity, the catalytic activity and stability are interrelated and bridged by the Ru-O bonding nature, i.e. bond covalency and level of difficulty in Ru-O bond breaking [50] , as follows. Weakening the Ru-O bond covalency implies the burying of the O 2 p orbital under the Fermi level as well as the Ru 3 d front orbital, thereby prohibiting lattice oxygen from participating in OER and the formation of oxygen vacancy (Δ G VO ) [45] , [51] . In thus formed catalysts dominated by AEM, too low degree of Ru-O hybridization indicates too weak oxygen binding strength, which causes decreased Ru vacancy formation energy (Δ G VRu ) and eases Ru loss [52] , resulting in a simultaneous decrease in activity and stability. Strengthening the Ru-O bonding will firstly lead to a moderate intermediate binding energy as well as an increased Δ G VRu under AEM, thereby improving both the activity and stability [53] , [54] . However, further increasing the bonding strength leads to arise of lattice oxygen redox, where O 2 p becomes the front orbital and thereby causes lowered Δ G VO value [18] . Such a condition, though greatly boosts the intrinsic activity, causes the formation of oxygen defects and easy detachment of Ru-Ox moieties from defects' neck, leading to rapid catalyst degradation [28] , [37] . To this end, an appropriate performance indicator might be a physical parameter that could precisely describe the local Ru-O bonding nature. We postulate that the Ru charge might be able to serve as such an intuitive descriptor, because it could not only perfectly reflect the local Ru-O bonding structure, i.e., the ionic or covalent bonding, but also the bonding strength. Therefore, it is possible to customize both the reaction activity and stability, using Ru charge as a regulator (Fig. 1 ). We, therefore, begin our study by looking for a suitable model catalyst system to verify this idea, and found that the MRuO x solid solution (M in +4 valence to avoid additional structure influence) with a clear Ru-O-M structure motif might be suitable for such a proposal. Specifically, the Ru charge can be regulated by adjusting the ionic electronegativity of M, where M 4+ in higher ionic electronegativity than Ru 4+ leads to reduced electron density on Ru, and vice versa. Consequently, we selected M = Ce 4+ , Sn 4+ , Ru 4+ , and Cr 4+ with an ionic electronegativity of 1.608, 1.706, 1.848, and 1.861 to carry out our further study [55] , [56] . Fig. 1: Relation between catalytic performance and Ru charge. Schematic illustration of OER activity and stability of Ru-based catalysts within different reaction routes on the scale of Ru charge. Full size image DFT calculational predictions We firstly carried out DFT calculations with the simulation model of M 0.5 Ru 0.5 O 2 with Ru-O-M motifs constructed (Fig. 2a ) based on the stable rutile RuO 2 (110) [18] , [57] (Supplementary Figs. 2 – 6 and Supplementary Note 1 ). The charge of Ru in Ru-O-M was first calculated. As the electronegativity of M 4+ increases from 1.608 (Ce 4+ ) to 1.861 (Cr 4+ ), the charge of Ru increased from 1.49 (Ce 0.5 Ru 0.5 O 2 ) to 1.57 (Cr 0.5 Ru 0.5 O 2 ) (Fig. 2b ). We then evaluated the dependence of theoretical OER activity on the Ru charge, in both AEM and LOM reaction pathways on Ru sites, as the M sites were calculated to possess extremely poor activities under both reaction pathways (M = Ce, Sn, Cr) (Supplementary Figs. 7 – 13 and Supplementary Note 2 ). Fig. 2: Prediction of the OER performance based on DFT calculation. a Schematics of two OER pathway (AEM and LOM) on the surface of M 0.5 Ru 0.5 O 2 (110). b The variation of Ru charge in M 0.5 Ru 0.5 O 2 with an ionic electronegativity of different M. c Theoretical overpotential volcano plot under AEM pathway as a function of the Ru charge. d Projected DOS plots of Ru ( d ) and O ( p ) near the Fermi level for M 0.5 Ru 0.5 O 2 . The light gray filling shows the overlap between Ru ( d ) and O ( p ). e Variation of O ( p ) contribution near Fermi level with Ru charge. f Theoretical overpotential plot under LOM pathway as a function of the Ru charge. g The Ru vacancy formation energy (Δ G VRu ) of M 0.5 Ru 0.5 O 2 is characterized by Ru charge. For RuO 2 and Cr 0.5 Ru 0.5 O 2 , Δ G VRu were calculated without (transparent dots in yellow and green) and with (opaque dots in yellow and green) the consideration of lattice oxygen vacancies. Source data are provided as a Source Data file. Full size image The AEM pathway activities of the materials are revealed to follow a volcanic-like trend as a function of Ru charge. The theoretical OER overpotentials of M 0.5 Ru 0.5 O 2 were calculated first, with the Sn 0.5 Ru 0.5 O 2 sample exhibiting moderate Ru charge (1.52) representing the lowest theoretical OER overpotential. For the samples with both lower (Ce 0.5 Ru 0.5 O 2 ) and higher (RuO 2 and Cr 0.5 Ru 0.5 O 2 ) Ru charge, increases in OER overpotentials are observed (Fig. 2c and Supplementary Figs. 14 – 17 ). While this phenomenon implies that an optimum Ru charge that is neither too high nor too low is beneficial for OER, the underlying reason is that Ru charge can be successfully used to reflect the Ru-O bonding interaction. Specifically, we calculated the overlap band center of Ru d orbital and O p orbital in the partial density of states (pDOS, Supplementary Fig. 18 ) [58] and found that the overlap band center (ε-Ru d -O p ) takes the same trending with the change in Ru charge, i.e., increases from −4.19 to −2.95 eV with an increase in Ru charge (1.49–1.57). To this end, the Ru charge can truly be utilized as the intuitive descriptor because it reflects the status of both Ru itself and the Ru-O orbital interaction. Indeed, as the Ru charge increases, the M 0.5 Ru 0.5 O 2 undergoes alteration in the potential determine step (PDS) from OH*/O* to O*/OOH* (Supplementary Figs. 13 , 14 ), due to strengthening in Ru-O* binding, in line with bond shrinkage from 1.749 to 1.732 Å (Supplementary Fig. 19 ). Therefore, Ru sites charge can be successfully used to indicate the AEM reaction activity. We then move to calculate the reactivity of lattice oxygen in different M 0.5 Ru 0.5 O 2 structures and the feasibility of the LOM route. First, upshifting in O 2 p band center (Fig. 2d, e and Supplementary Fig. 20 ) and strengthening in Ru-O bond covalency are observed with increases in Ru charge, as indicated by increases in both ε-O p -Ru d , O 2 p band contribution near the E F (from 2.2 to 25.2%) [40] , [59] , [60] and downshifted ICOHP between Ru and O (from −1.280 to −1.733 eV, Supplementary Figs. 21, 22 ). Second, we calculated the formation energies of oxygen vacancy(Δ G VO ) in different samples, to analyze the occurrence possibility of LOM [18] . The significantly downshifted Δ G VO from 7.20 eV (Ce 0.5 Ru 0.5 O 2 ) and 8.25 eV (Sn 0.5 Ru 0.5 O 2 ) to 5.68 eV (RuO 2 ) and 5.29 eV (Cr 0.5 Ru 0.5 O 2 ) suggests the higher possibility of LOM involvement in RuO 2 and Cr 0.5 Ru 0.5 O 2 with high Ru charge (Supplementary Fig. 23 ). The lower Δ G VO of Ce 0.5 Ru 0.5 O 2 compared to that of Sn 0.5 Ru 0.5 O 2 may originate from the distortion of the crystal structure [61] (Supplementary Figs. 24 – 27 and Supplementary Note 3 ). Third, we turned to calculate the LOM energy variation for M 0.5 Ru 0.5 O 2 (Fig. 2f and Supplementary Figs. 28 – 31 ). Clearly, the theoretical overpotential of OER under the LOM path gradually decreases from 0.84 V for Ce 0.5 Ru 0.5 O 2 to 0.34 V for Cr 0.5 Ru 0.5 O 2 . Therefore, the direct O-O coupling on the O p band above the E F is more thermodynamically favored with a higher Ru charge (i.e., in RuO 2 and Cr 0.5 Ru 0.5 O 2 ). Based on the above calculations, the correlation between a charge of the Ru site and the reaction path (AEM and LOM) as well as reaction energy on M 0.5 Ru 0.5 O 2 (Fig. 1 ) is unveiled. While low charge (Ce 0.5 Ru 0.5 O 2 and Sn 0.5 Ru 0.5 O 2 ) at Ru sites leads to the domination of the AEM path, the LOM route is energetically more favored at elevated Ru charge. Moreover, by changing the Ru charge, the OER catalytic activity of catalysts following AEM can also be adjusted due to the regulation of Ru-O interaction in M 0.5 Ru 0.5 O 2 . We then move to our next step, i.e., probing the applicability of the Ru charge in describing the stability of the catalysts. Two indicators, i.e., the formation energies of Ru (Δ G VRu ) and O (Δ G VO ) vacancies, are used jointly to describe the stability of the catalysts. On one hand, it is expected that increasing the Ru charge results in strengthened Ru-O bonding and thereby increased Δ G VRu in perfectly crystallized M 0.5 Ru 0.5 O 2 samples, with Δ G VRu increasing gradually from 9.44 eV in Ce 0.5 Ru 0.5 O 2 to13.92, 14.60, and 15.13 eV for Sn 0.5 Ru 0.5 O 2 , RuO 2 , and Cr 0.5 Ru 0.5 O 2 , respectively (Fig. 2g ). On the other hand, however, increase in Ru charge causes ease formation of O V (Supplementary Fig. 23 ) and thereby decreases in Δ G VRu (Supplementary Fig. 32 ) due to lower overall Ru-O chelation number. Specifically, with the formation of one neighboring O V , the Δ G VRu value for RuO 2 and Cr 0.5 Ru 0.5 O 2 decreases from 14.60 and 15.13 eV to 8.51 and 7.95 eV, respectively, resulting in poor stability (Fig. 2g ). To this end, the Sn 0.5 Ru 0.5 O 2 near the apex of the volcano curve under the AEM path demonstrates the best stability. The rationale behind this is that the low Ru charge (Ce 0.5 Ru 0.5 O 2 ) makes the Ru species prone to dissolution in acid, too high Ru charge leads to the readily generation of O V defects and smaller Δ G VRu , thus resulting in the overall destabilization. Since metal dissolution may occur during acidic OER, defective structures with Ru and M vacancies were also constructed for calculations (Supplementary Figs. 33 – 43 and Supplementary Note 4 ). Although the inclusion of metal center vacancies leads to the trend of crossover between AEM and LOM pathways (Supplementary Fig. 44 ), in line with recent work from Alexandrov et al. [62] , [63] , Ru charge is still valid in describing the reaction path and energy as the vacancies influence the Ru charge and OER reaction in the same way. Specifically, the inclusion of vacancies leads to the evolution of the Ru-O bonding feature and thereby Ru charge (Supplementary Fig. 45 and Supplementary Note 5 ), which thus determines the theoretical activity under different paths. As a result, the theoretical performance of defective M 0.5 Ru 0.5 O 2 on the scale of Ru charge perfectly matches that of the non-defective structure. To here, it is clear that the Ru charge can be used to describe not only the major reaction path and OER activity, but also the structural stability, due to its successful reflection in both electronic features of Ru and overall Ru-O bonding interactions (Fig. 1 ). Synthesis and characterization To experimentally validate the DFT prediction, MRuO x oxide solid solution with a M/Ru ratio close to 1 was synthesized according to the previous reports (see Methods for details) [16] , [35] . Powder X-ray diffraction (XRD) patterns show that all prepared MRuO x samples possess a rutile-type structure without any distinct diffraction peaks corresponding to MO x and RuO 2 (Supplementary Fig. 46 ), indicating the formation of MRuO x oxide solid solution, in line with the uniform elements distribution revealed by energy-dispersive X-ray spectroscopy (EDX) (Supplementary Figs. 47 – 50 ). Rietveld refinement analysis (Supplementary Fig. 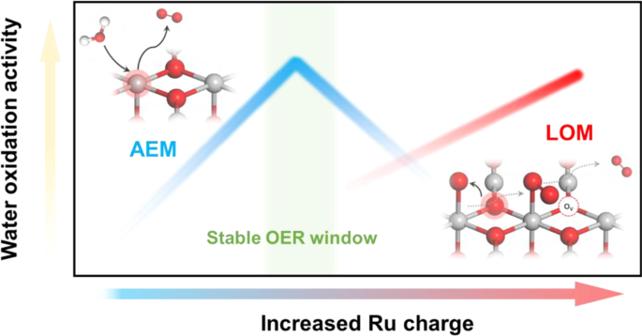Fig. 1: Relation between catalytic performance and Ru charge. Schematic illustration of OER activity and stability of Ru-based catalysts within different reaction routes on the scale of Ru charge. 51 and Supplementary Table 1 ) suggests the random displacement of Ru by M in MRuO x solid solution, giving the formation of Ru-O-M structure motif (Supplementary Fig. 52 ). The atomic ratios of M and Ru were close to 1, as analyzed by inductively coupled plasma optical emission spectrometer (ICP-OES) and EDX (Supplementary Fig. 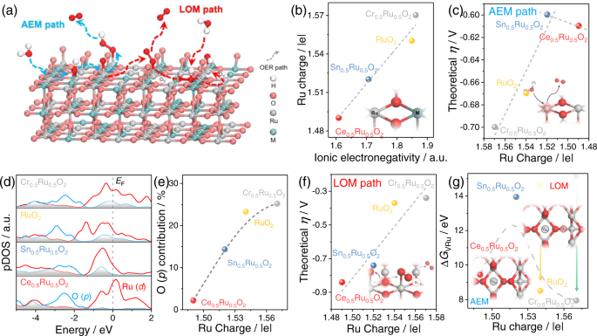Fig. 2: Prediction of the OER performance based on DFT calculation. aSchematics of two OER pathway (AEM and LOM) on the surface of M0.5Ru0.5O2(110).bThe variation of Ru charge in M0.5Ru0.5O2with an ionic electronegativity of different M.cTheoretical overpotential volcano plot under AEM pathway as a function of the Ru charge.dProjected DOS plots of Ru (d) and O (p) near the Fermi level for M0.5Ru0.5O2. The light gray filling shows the overlap between Ru (d) and O (p).eVariation of O (p) contribution near Fermi level with Ru charge.fTheoretical overpotential plot under LOM pathway as a function of the Ru charge.gThe Ru vacancy formation energy (ΔGVRu) of M0.5Ru0.5O2is characterized by Ru charge. For RuO2and Cr0.5Ru0.5O2, ΔGVRuwere calculated without (transparent dots in yellow and green) and with (opaque dots in yellow and green) the consideration of lattice oxygen vacancies. Source data are provided as a Source Data file. 53 and Supplementary Table 2 ). We then move on to probe the local structure and chemical states of Ru and O in MRuO x . X-ray photoelectron spectra (XPS) show that both Ru 3 d and Ru 3 p 3/2 (Fig. 3a ) signals could be deconvoluted into two doublets, representing Ru 4+ (fill in green) and the satellite peaks (fill in yellow) [54] , [64] . Notably, the Ru 3 d and Ru 3 p binding energies for CeRuO x (280.1 and 461.9 eV), SnRuO x (280.4 and 462.1 eV), RuO x (280.6 and 462.5 eV), and CrRuO x (280.8 and 462.8 eV) consecutively shifted to more positive values, implying a successive increase in Ru valence states, in line with the DFT calculation results. We further collected the Ru K edge spectra through X-ray absorption near-edge spectroscopy (XANES) to quantitatively describe the oxidation state of Ru. As presented in Fig. 3b , taking Ru foil and commercial RuO 2 as references, the oxidation states of Ru in MRuO x were estimated to be +3.3, +3.6, +3.9, and +4.2 for CeRuO x , SnRuO x , RuO x , and CrRuO x , respectively. The variation in Ru valence and its consistency with DFT calculation results verifies the feasibility of tailoring the Ru electron density via controlling the element M in the Ru-O-M motif, making it promising for reaction path and O* adsorption energy regulation. Fig. 3: Structure properties of MRuO x oxide solid solution experimentally obtained. a High-resolution Ru 3 d and Ru 3 p 3/2 XPS pattern of MRuO x , demonstrating the variation of Ru chemical states. b Ru K edge XANES spectra and corresponding first derivative (insert in the left part of b ) of MRuO x , Ru foil, and oxidized commercial RuO 2 . The right part of b show the relation between the Ru K -edge absorption energy ( E 0 ) and oxidation states for MRuO x and reference samples. c Ru L 3 -edge XAS spectra and the corresponding second derivative (insert in the left part of c ) of MRuO x . The right part of c illustrated the relation between the energy splitting Δ E and Ru oxidation states of MRuO x . d DEMS signals of 32 O 2 ( 16 O 16 O), 34 O 2 ( 16 O 18 O), and 36 O 2 ( 18 O 18 O) from the reaction products for MRu 16 O x in H 18 O aqueous sulfuric acid electrolyte. The right part of d presented the variation of the 16 O: 18 O ratio with Ru oxidation states of MRuO x . The dashed lines in c and d are used to guide the eyes. Source data are provided as a Source Data file. Full size image We next turned to validate experimentally if the OER path of MRuO x truly follows the DFT calculation results as a function of Ru charge, initiated by monitoring the Ru-O bond covalency via Ru XANES spectrum at L 3 edge (Fig. 3c ) [65] . As reported previously, the Ru XANES spectrum at the L 3 edge can be fitted by two peaks ascribable to e g and t 2g , and the energy splitting Δ E (Δ E = E e g - E t 2g ) is positively correlated with the Ru-O bond covalency. Notably, we find that Δ E increases from 1.51 to 1.95 eV (Fig. 3c , right) with the increase in valence state (+3.3 to +4.2), thus testifying to the greatly enhanced Ru-O bond covalency with increased Ru charge, in line with the increase in Ru d –O p overlap in the calculation (Fig. 2d, e ). O 1 s XPS spectra (Supplementary Fig. 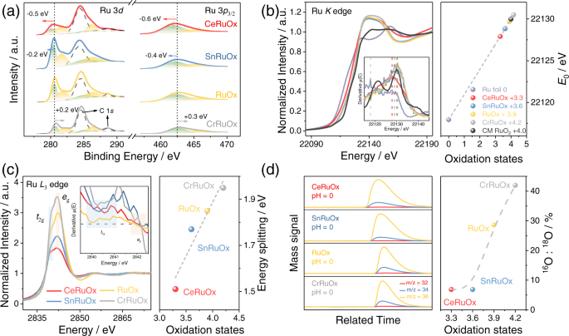Fig. 3: Structure properties of MRuOxoxide solid solution experimentally obtained. aHigh-resolution Ru 3dand Ru 3p3/2XPS pattern of MRuOx, demonstrating the variation of Ru chemical states.bRuKedge XANES spectra and corresponding first derivative (insert in the left part ofb) of MRuOx, Ru foil, and oxidized commercial RuO2. The right part ofbshow the relation between the RuK-edge absorption energy (E0) and oxidation states for MRuOxand reference samples.cRuL3-edge XAS spectra and the corresponding second derivative (insert in the left part ofc) of MRuOx. The right part ofcillustrated the relation between the energy splitting ΔEand Ru oxidation states of MRuOx.dDEMS signals of32O2(16O16O),34O2(16O18O), and36O2(18O18O) from the reaction products for MRu16Oxin H18O aqueous sulfuric acid electrolyte. The right part ofdpresented the variation of the16O:18O ratio with Ru oxidation states of MRuOx. The dashed lines incanddare used to guide the eyes. Source data are provided as a Source Data file. 54 and Supplementary Table 3 ) further suggest significant increases in O V contents in RuO x (36%) and CrRuO x (41%) compared with that of CeRuO x (25%) and SnRuO x (15%), in good compliance with the increase in bond covalency [11] . The occurrence of LOM is further verified by in situ 18 O isotope-related DEMS measurements on all MRuO x samples (Fig. 3d , Supplementary Figs. 55 – 63 , and Supplementary Note 6 ) according to the previous reports [66] , [67] , [68] . By extrapolating the integration of the mass spectra signal ( 16 O/ 18 O) per second to the OER onset, the content of the LOM path during OER is determined (Supplementary Figs. 55 – 63e ). Specifically, the AEM path is revealed to be dominant on CeRuO x and SnRuO x , as the 16 O/ 18 O ratio of O 2 catalyzed by CeRu 16 O x and SnRu 16 O x in 18 O-labeled 0.5 M H 2 SO 4 is 6.88 and 6.85% (Supplementary Figs. 56 , 57e ), respectively, which is consistent with that of the commercial IrO 2 (6.56%, Supplementary Fig. 55 ), attributable to the isotopic abundance of 16 O in H 2 18 O. On Ru 18 O x and CrRu 18 O x , however, the 16 O/ 18 O ratio in products significantly increased to 28.63 and 41.96%, leading to an increment in the LOM ratio of RuO x and CrRuO x to 12.6 and 36.7%, respectively (Supplementary Figs. 58 – 59 ). Besides, the DEMS measurements in 18 O-labeled 0.1 M PBS (pH = 6) also demonstrate similar results (Supplementary Figs. 60 – 63 ). It is noted that the LOM ratio differs significantly in literature as reported by refs. [67] , [68] , [69] , etc., mainly owing to the difference in structural properties of the catalysts, while our result is in high accordance with that reported by ref. [38] , due to the similar solid solution structure (Supplementary Note 7 ). To here, it is clear that the Ru charge is a useful parameter to customize the OER path on MRuO x . OER catalytic performance in a three-electrode configuration The OER performance of the prepared MRuO x was firstly evaluated in a conventional three-electrode setup at a catalyst loading of 41.65 μg cat cm −2 (Supplementary Figs. 64, 65 and Supplementary Note 8 ) with 0.5 M H 2 SO 4 electrolyte according to the guideline recently set [70] , [71] . The linear sweep voltammetry (LSV) curves normalized by the geometric area (Fig. 4a ), electrochemical active surface area (ECSA) (Supplementary Fig. 66a, b ), Ru mass loading on the electrode (Supplementary Fig. 66c ) and corresponding Tafel slopes (Supplementary Fig. 66d–f ) revealed the variation in OER catalytic activity of MRuO x . As summarized in Fig. 4b and Supplementary Fig. 67 , the activity trend of MRuO x is in good agreement with DFT prediction. Specifically, on samples dominated by AEM path (CeRuO x and SnRuO x ), the OER activity is significantly enhanced with an increase in Ru charge (strengthened O* adsorption), accompanied by the variation in reaction determine step as indicated by the difference in Tafel slope (60.2 and 38.2 mV dec −1 ) (Supplementary Fig. 66d and Supplementary Note 9 ). Further increase in the Ru charge leads to a performance decline in AEM but the occurrence of LOM. Therefore, an activity drop in RuO x and a slight lift in CrRuO x are observed, in line with the DFT calculation. Notably, the SnRuO x customized near the apex of AEM exhibited remarkable OER catalytic activity. Satisfactorily, a small catalytic overpotential ( η ) of 194 mV is needed for SnRuO x to deliver a current density of 10 mA cm −2 , which is 176 mV lower than that of commercial RuO 2 (Fig. 4a ). Furthermore, the mass activity and turnover frequency (TOF) of SnRuO x at 1.48 V vs. RHE is 36.4 times that of commercial RuO 2 , reaching 2360 A g Ru −1 and 0.63 s −1 (Supplementary Fig. 68 ). These results unambiguously suggest SnRuO x as one of the most active Ru-based catalysts towards acidic OER (Fig. 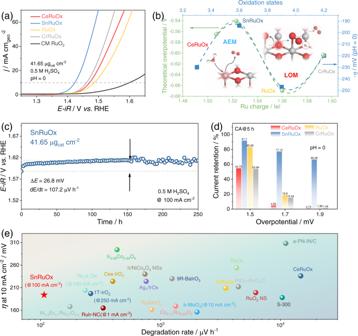Fig. 4: Electrocatalytic performance of MRuOxin three-electrode setup. aGeometric area normalized LSV curves of MRuOx.bThe variation of apparent overpotential at 10 mA cm−2with Ru oxidation states. The theoretical overpotential of MRuOxis the weighted value of the theoretical activity of different reaction mechanisms to its proportions (from Supplementary Fig.56-59). The apparent overpotential experimentally obtained is given as the blue dots scaled with the right Y-axis. The theoretical overpotential is given as the green dots scaled with the left Y-axis.cChronopotentiometry curve of SnRuOxnanocatalyst operated at 100 mA cm−2during the 250 h test.dCurrent retention of MRuOxafter chronoamperometry test at various potentials (1.5 V, 1.7 V, and 1.9 V) for 5 h.eComparison of OER performance (ηat 10 mA cm−2and activity degradation rate) for variously reported electrocatalysts. SnRuOxis presented by a red star. The electrocatalytic performance is collected with a catalyst loading of 41.65 μgcatcm−2. Source data are provided as a Source Data file. 4e and Supplementary Table 4 ). Fig. 4: Electrocatalytic performance of MRuO x in three-electrode setup. a Geometric area normalized LSV curves of MRuO x . b The variation of apparent overpotential at 10 mA cm −2 with Ru oxidation states. The theoretical overpotential of MRuO x is the weighted value of the theoretical activity of different reaction mechanisms to its proportions (from Supplementary Fig. 56 - 59 ). The apparent overpotential experimentally obtained is given as the blue dots scaled with the right Y-axis. The theoretical overpotential is given as the green dots scaled with the left Y-axis. c Chronopotentiometry curve of SnRuO x nanocatalyst operated at 100 mA cm −2 during the 250 h test. d Current retention of MRuO x after chronoamperometry test at various potentials (1.5 V, 1.7 V, and 1.9 V) for 5 h. e Comparison of OER performance ( η at 10 mA cm −2 and activity degradation rate) for variously reported electrocatalysts. SnRuO x is presented by a red star. The electrocatalytic performance is collected with a catalyst loading of 41.65 μg cat cm −2 . Source data are provided as a Source Data file. Full size image We then tested the stability of MRuO x during operation to probe into the effectiveness of Ru charge in describing the stability. To start with, chronoamperometry (CA) tests (5 h) suggest SnRuO x as the most stable catalyst, with high current retention of 91.7, 77.15, and 66.48% after operating at 1.5, 1.7, and 1.9 V vs. RHE, respectively (Supplementary Fig. 69 ). By contrast, the CeRuO x , CrRuO x , and RuO x only demonstrate current retention of 54.75, 83.09, and 53.84% at 1.5 V vs. RHE, respectively, implying their poor stability. Furthermore, to eliminate the interference of other factors beyond the catalyst, i.e., thin film quality [72] , [73] , active sites blockage [74] , and back electrode passivation [75] , [76] , the stability of MRuO x was evaluated by monitoring the dissolution behavior of M and Ru during CA tests. By calculating the Ru stability number (S-number) [77] during CA tests, the stability of MRuO x is found to be in line with the Δ G VRu from the DFT calculations (Supplementary Fig. 70 ). Given the perfect match in catalytic stability between experiments and theoretical computations, we further run a CP test at 100 mA cm −2 for the SnRuO x sample to verify its stability (Fig. 4c ). 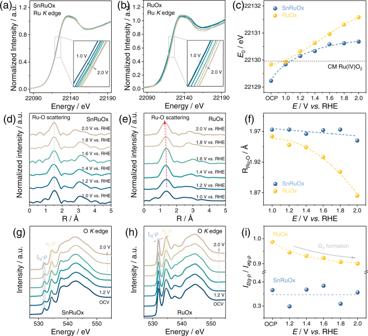Fig. 5: Investigating the stability mechanism of SnRuOxduring OER with RuOxas control. a,bIn situ RuKedge XANES spectra of SnRuOx(a) and RuOx(b) with applied bias rise from 1.0 V to 2.0 V vs. RHE.cThe variation trend of RuK-edge absorption energy (E0) of SnRuOxand RuOxunder different potentials.d,eFourier transforms ofk2-weighted EXAFS signals of SnRuOx(d) and RuOx(e) with applied bias rise from 1.0 to 2.0 V vs. RHE.fSummary of the Ru-O bond length of SnRuOxand RuOxunder various potentials according to the quantitative fitting results (Supplementary Table7).g,hQuasi in situ OKedge XAS TEY spectra of SnRuOx(g) and RuOx(h) with an applied potential increase from 1.2 to 2.0 V vs. RHE.iThe variation ofIt2g-p/Ieg-pwith applied potential for SnRuOxand RuOx. The dashed lines inc,f,iare used to guide the eyes. Source data are provided as a Source Data file. 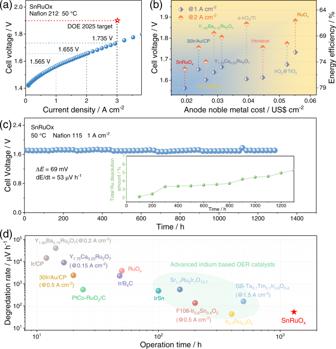Fig. 6: Performance of PEM electrolyzer using SnRuOxas anode electrocatalyst. aPolarization curve of the PEM electrolyzer obtained at 50 °C with Nafion 212 membrane.bComparison of the efficiency of previously reported anode electrocatalysts. The X-axis represents the anode noble metal cost (Supplementary Table8). The left and right Y-axis represent the cell voltage and energy efficiency at 1 and 2 A cm−2respectively.cChronopotentiometry curve of the PEM electrolyzer using SnRuOxcatalyst operated at 1 A cm−2at 50 °C with Nafion 115 membrane. Insert incshow the total dissolution amount of Ru during the 1300 h test.dComparison of the operational stability (operation time and performance degradation rate) of SnRuOxwith reported anode catalysts. Source data are provided as a Source Data file. Excitingly, during a 250 h test, the overpotential only increased by 26.8 mV, giving a degradation rate of merely 107.2 μV h −1 , three orders of magnitude smaller than that of commercial RuO 2 (Supplementary Fig. 71 ) and comparable to that of the advanced Ir-based catalysts (Fig. 4e and Supplementary Tables 5 , 6 ) [12] , [14] , [18] , [19] , [38] , [52] , [53] , [54] , [78] , [79] , [80] , [81] , [82] , [83] , [84] , [85] , [86] , [87] , [88] , [89] , [90] . Besides, by carrying out CA tests in a weak acidic environment (0.1 M PBS, pH = 6), the contribution of M (M = Ce, Sn, and Cr) dissolution on the performance degradation of MRuO x is eliminated (Supplementary Figs. 72 , 73 and Supplementary Note 10 ), further demonstrating the stability of MRuO x is dependent on the Ru stability. These results corroborate the effectiveness of the Ru charge not only in describing the trend in catalytical activity, but more importantly, in screening out the most durable catalysts ever reported. The origin of the high stability To further probe into the stabilization mechanism of SnRuO x during OER operation, we adopted in situ XAS and in situ Raman spectroscopy to investigate the dynamic variation in local Ru structure and chemical environment. RuO x was also tested as the counterpart catalyst for comparison. According to the literature, the over-oxidation of Ru originating from the structure damage under high oxidation potential is one of the main culprits leading to severe Ru dissolution [91] . Thus, Ru K edge XANES spectra were collected to monitor the change in Ru oxidation states of SnRuO x and RuO x during operation. As presented in Fig. 5a, b and summarized in Fig. 5c , SnRuO x and RuO x show big differences in Ru valence states during operation (Supplementary Fig. 74 ), especially at higher applied potentials. Specifically, switching on the electrode potential from open circuit potential (OCP) to 1.4 V vs. RHE leads to a rapid rise in Ru valence from +3.6 to +4.2 in SnRuO x , followed by a gentle and steady change from +4.2 to +4.4 with potential further lifted to 2.0 V vs. RHE. On the contrary, the Ru oxidation states in RuO x increase at a constant rate from +3.9 to +4.9 with the applied potential ranging from OCP to 2.0 V vs. RHE, showing no sign of stabilization. This result indicates that even at high oxidation potentials, the stable structure of SnRuO x can be maintained under the customized AEM path, whereas RuO x undergoes significant structural evolution, probably ascribable to the involvement of LOM. Fig. 5: Investigating the stability mechanism of SnRuO x during OER with RuO x as control. a , b In situ Ru K edge XANES spectra of SnRuO x ( a ) and RuO x ( b ) with applied bias rise from 1.0 V to 2.0 V vs. RHE. c The variation trend of Ru K -edge absorption energy ( E 0 ) of SnRuO x and RuO x under different potentials. d , e Fourier transforms of k 2 -weighted EXAFS signals of SnRuO x ( d ) and RuO x ( e ) with applied bias rise from 1.0 to 2.0 V vs. RHE. f Summary of the Ru-O bond length of SnRuO x and RuO x under various potentials according to the quantitative fitting results (Supplementary Table 7 ). g , h Quasi in situ O K edge XAS TEY spectra of SnRuO x ( g ) and RuO x ( h ) with an applied potential increase from 1.2 to 2.0 V vs. RHE. i The variation of I t 2g- p / I e g- p with applied potential for SnRuO x and RuO x . The dashed lines in c , f , i are used to guide the eyes. Source data are provided as a Source Data file. Full size image We then carried out in situ Raman spectroscopy to clarify the structure evolution during OER. For both SnRuO x and RuO x , two major peaks at ~435 and 595 cm −1 assignable to E g and A 1g vibration modes were observed (Supplementary Fig. 75 ) [92] , [93] . With the potential increases from OCP to 1.8 V vs. RHE, the SnRuO x sample maintains a constant Raman shift, suggesting the consistency in Ru-O bonding structure during OER. However, a ca . 9 cm −1 positive shift in RuO x is noticed, implying the shrinkage in Ru-O bonding length during OER. To intuitively uncover the local structure evolution of SnRuO x and RuO x during OER, Fourier transforms (FTs) analysis of extended X-ray absorption fine structure (EXAFS) spectra was carried out to provide R -space information. A prominent peak of ~1.45 Å (phase uncorrected) corresponds to the first Ru-O coordination shell can be observed (Fig. 5d, e and Supplementary Figs. 76, 77 ) for both samples. Interestingly, while only small fluctuations in Ru-O bond length (r Ru-O ) are observed for SnRuO x (from 1.97 to 1.96 Å) with potential increases from 1.0 to 2.0 V vs. RHE, a significant r Ru-O shrinkage from 1.96 to 1.86 Å is observed in RuO x (Fig. 5f ), in well accordance with the Raman results. Meanwhile, while quantitative Ru K edge fitting results (Supplementary Table 7 ) show no significant change in Ru-O coordination number (CN) for SnRuO x , a significant decrease in CN from 6.4 to 4.7 is evidenced in RuO x , ascribable to the generation of O V due to the occurrence of LOM. We further performed quasi in situ soft-XAS measurements to collect the O K edge information, to directly evidence the formation of O V by recording the total electron yield (TEY) intensity before and after operating under different potentials. Two pre-edge peaks at ~532 and 534.5 eV assignable to the unoccupied orbital of O 2 p hybridized with Ru 4 d t 2g and e g orbitals are observed for both SnRuO x and RuO x (Fig. 5g–i ) [45] . According to previous reports, the reduction in t 2g - p / e g - p peak intensity ( I t 2g- p / I e g- p ) implies the formation of the O V due to the electron occupation of the lowest energy state ( t 2g ) of octahedral symmetry [94] , [95] . For RuO x , the ratio of I t 2g- p / I e g- p decreases monotonously with potential increases from 1.2 to 2.0 V vs. RHE, implying the generation of a high amount of O V during OER. On the contrary, no obvious variation in I t 2g- p / I e g- p is observed for SnRuO x , suggesting that there is no increase in O V content and thus ruling out the occurrence of LOM, which endows it with excellent operational stability. These results are in good agreement with the catalyst design idea as SnRuO x was customized to follow the AEM path and exhibited high stability during OER due to moderate Ru charge. Performance of PEMWE devices Encouraged by the overall high activity and stability of SnRuO x towards OER, we finally assembled a single cell using the catalyst as the anode to evaluate its performance in a real PEMWE device (Supplementary Fig. 78 , see Methods for details). The steady-state polarization curve of membrane electrode assemblies (MEAs) operated at 50 °C (Fig. 6a ) shows that the performance of PEMWE can be greatly improved with the utilization of SnRuO x . Specifically, cell voltages of only 1.565, 1.655, and 1.735 V are needed to reach current densities of 1, 2, and 3 A cm −2 , respectively, far superior to that obtained with commercial RuO 2 (1.733 V@1 A cm −2 and 1.883 V@2 A cm −2 ) (Supplementary Fig. 79 ) and also well surpassing the DOE 2025 target (3 A cm −2 @1.9 V) [96] . Taking noble metal cost and cell performance into account, the overall advantages of SnRuO x are self-evident (Fig. 6b ). With anode noble metal cost of US$ 0.0194 cm −2 , high energy efficiencies at 78.7 and 74.3% were achieved at 1 and 2 A cm −2 , respectively, corresponding to energy consumptions at 41.9 and 44.4 kWh kg −1 H 2 , outperforming the prior reported most cost-efficient OER catalysts (Fig. 6b , Supplementary Table 8 , and Supplementary Note 11 ) [20] , [97] , [98] , [99] , [100] , [101] , [102] . According to the calculation from US DOE, only US$ 0.838 is required for this PEMWE device to produce 1 kg H 2 , which is much lower than the DOE target (<US$2 kg H2 −1 ), further proving the efficiency of the SnRuO x at the anode. Fig. 6: Performance of PEM electrolyzer using SnRuO x as anode electrocatalyst. a Polarization curve of the PEM electrolyzer obtained at 50 °C with Nafion 212 membrane. b Comparison of the efficiency of previously reported anode electrocatalysts. The X-axis represents the anode noble metal cost (Supplementary Table 8 ). The left and right Y-axis represent the cell voltage and energy efficiency at 1 and 2 A cm −2 respectively. c Chronopotentiometry curve of the PEM electrolyzer using SnRuO x catalyst operated at 1 A cm −2 at 50 °C with Nafion 115 membrane. Insert in c show the total dissolution amount of Ru during the 1300 h test. d Comparison of the operational stability (operation time and performance degradation rate) of SnRuO x with reported anode catalysts. Source data are provided as a Source Data file. Full size image The long-term operational stability is even more exciting, as shown in Fig. 6c , the SnRuO x -based cell demonstrates well-maintained PEMWE performance after running under 1 A cm −2 for 1300 h, with apparent degradation rate only at 53 μV h −1 . Such stability not only represents a record for Ru-based catalysts, but even superior to that of the advanced Ir-based OER catalysts recently reported (Fig. 6d and Supplementary Table 9 ) [14] , [20] , [38] , [52] , [97] , [99] , [103] , [104] , [105] , [106] , [107] . To more accurately determine the lifetime of SnRuO x in PEMWE, a modified MEA setup without metallic parts in the anode and cathode water cycle was employed according to the previous reports (Supplementary Fig. 80 – 84 , Supplementary Table 10 , and Supplementary Note 12 ) [108] . With all the Ru dissolved in the anode/cathode water and membrane monitored during 10 h operation at 1 A cm −2 , the S-number of SnRuO x is calculated to be 1.04 × 10 6 (Supplementary Note 13 ) [77] . These results reveal the inherently robust nature of SnRuO x as an OER catalyst with highlighted practical application prospects. In summary, we presented a practical and feasible idea, namely customizing the reaction route, to design a highly active and stable Ru-based OER catalyst that can afford long-term operation in PEMWE devices. Based on the widely recognized OER mechanism, we found that Ru charge can be used as a scale for the reaction path of the catalyst, only those located close to the apex of the volcano plot in AEM can exhibit optimal stability. Subsequently, we verified the feasibility of this idea in an MRuO x model catalyst. By screening M 4+ with different ionic electronegativity, the Ru charge can be effectively regulated attributed to the charge redistribution effect in a Ru-O-M structure motif. As a result, the SnRuO x customized exhibited unparallel OER catalytic activity and stability. A PEMWE device assembled with SnRuO x as an OER catalyst can afford a cell voltage of only 1.565 V at 1 A cm −2 as well as long-term stability over 1300 h with a degradation rate of only 53 μV h −1 . This work provides a rational catalyst design concept at the level of reaction path customization, and provides a feasible solution for the practical application of Ir-free Ru-based catalysts in commercial PEMWE systems. Materials All chemicals were obtained from commercial suppliers at analytical grade and used as received without further purification. The commercial RuO 2 and Water− 18 O (H 2 18 O) were purchased from Aladdin. Carbon paper was obtained from Engineered Fibers Technology, LLC. Commercial Pt/C (40 wt% Pt) catalyst was purchased from Johnson Matthey Company. Titanium felt were purchased from Bekaert New Materials. 5 wt% Nafion® ionomer, Nafion 115 membrane, and Nafion 212 membrane were purchased from DuPont Co. The L shape gold electrode with an area of 0.07065 cm 2 is obtained from Tianjin Aida Hengsheng Technology Development Co., Ltd. Preparation of CeRuO x solid solution The CeRuO x solid solution was fabricated via a pyrolysis-thermal annealing strategy. Typically, glucose, RuCl 3 , and CeCl 3 ·7H 2 O were mixed and dried to obtain a xerogel with Ru and Ce uniformly distributed. Then the precursor was heated in air at 350 °C for 5 h with a heating rate of 5 °C min −1 . After cooling to room temperature, the collected samples were carefully ground and ultrasonically washed in 1 M HCl for at least 6 h to remove acid-labile components. Preparation of SnRuO x solid solution The SnRuO x solid solution was prepared following the procedure of ion exchange and thermal annealing. Firstly, an Sn-based metal-organic framework (MOF) was fabricated according to the previous reports. The ethanol solution of SnCl 4 and HMTA (Hexamethylenetetramine) is uniformly mixed and stirred at room temperature for 1 h, washed, and dried to obtain Sn-HMTA. Then Sn-HMTA were dispersed in the THF (Tetrahydrofuran) solution of RuCl 3 . After stirring for 24 h, the mixture is centrifuged and washed with THF to obtain an Sn/Ru-HMTA precursor. The dried products are conducted to heat treatment in air at 350 °C for 5 h with a heating rate of 5 °C min −1 . After cooling to room temperature, the collected samples were carefully ground and ultrasonically washed in 1 M HCl for at least 6 h to remove acid-labile components. Preparation of RuO x The preparation process of RuO x is similar to that of SnRuO x . The THF solution of RuCl 3 and HMTA was ultrasonically mixed and stirred at room temperature for 24 h, followed by centrifugation and washing. After drying in the oven, the Ru-HMTA precursor were annealed at 350 °C for 5 h with a heating rate of 5 °C min −1 in air. After cooling to room temperature, the collected samples were carefully ground and ultrasonically washed in 1 M HCl for at least 6 h to remove acid-labile components. Preparation of CrRuO x solid solution The CrRuO x solid solution were prepared according to the previous reports. The Cr, Ru containing precursors were obtained by mixing RuCl 3 and MIL-101(Cr) in THF and stirring for 24 h. The result RuCl 3 -MIL-101(Cr) were then heated to 450 °C and held for 5 h in air with a heating rate of 5 °C min −1 . After cooling to room temperature, the collected samples were carefully ground and ultrasonically washed in 1 M HCl for at least 6 h to remove acid-labile components. Structural characterizations Powder X-ray diffraction (XRD) patterns were collected using a Rigaku Smartlab diffractometer with Cu Kα radiation (λ = 1.5418 Å) in the scan range of 10° to 90° at a step of 0.01°. Scanning electron microscopy (SEM) measurements were performed on an XL 30 ESEMFEG field emission scanning electron microscopy. Transmission electron microscopy (TEM), high-resolution transmission electron microscopy (HRTEM), and elemental mapping analysis were performed on a Philips TECNAI G2 electron microscope operating at 200 kV. High-annular dark-field scanning transmission electron microscopy (HAADF-STEM) images were performed on a Titan 80-300 scanning/transmission electron microscopy operated at 300 kV. The surface electronic states were determined by X-ray photoelectron spectroscopy (XPS) using a Thermo Fisher Scientific ESCALAB 250Xi unit with Al-Kα (1486.6 eV) as the X-ray source. Inductively coupled plasma optical emission spectroscopy (ICP-OES; X Series 2, Thermo Scientific USA) was used to determine the ratio of M/Ru in the as-prepared samples and the dissolution of M and Ru after the stability tests. XAFS data collection and analysis The ex situ and in situ Ru K -edge XAFS measurements were performed at BL14W1 station in Shanghai Synchrotron Radiation Facility (SSRF, 3.5 GeV, 220 mA maximum, Si(111) double crystals). The Ru K -edge spectra of the samples were collected in transmission mode using a Lytle detector. The XAFS raw data were background-subtracted and normalized by the ATHENA program. Least-squares curve-fitting analysis of the EXAFS χ(k) data (including different coordination shells, in the R -space (1.0−3.0 Å)) and Fourier transforms (in the k -space 3.1−11.0 Å −1 ) were carried out using the ARTEMIS program. The theoretical scattering amplitudes, phase shifts, and the photoelectron mean free path for all paths were calculated by using a Hanning window (d k = 1.0 Å −1 ) in the IFEFFIT package. The data were fitted in R -space with theoretical models constructed on the basis of the crystal structure derived from XRD. The ex situ Ru L 3 edge measurements were carried out at the soft X-ray microcharacterizaiton beamline (SXRMB) in Canadian Light Source (CLS). The O K edge XAFS was measured at the BL08U1A beamline, SSRF. Electrochemical measurements in a three-electrode cell The electrochemical performance of the as-prepared catalysts were measured in a standard three-electrode cell on PARSTAT MC (AMETEK®). The electrocatalysts (1 mg) were dispersed in a mixture of 0.890 mL ethanol, 100 μL ethylene glycol, and 10 μL Nafion® solution (5 wt%). The ethylene glycol is introduced to improve the quality of the catalyst thin film and suppress the coffee-ring effect according to the previous work from ref. [6] . After ultrasonication for 1 h, the desired amount of homogeneous ink was dropped on a polished L shape gold electrode (area 0.07065 cm −2 ) and dried in an oven (60 °C) for 30 min and then serve as a working electrode. After loading optimization, the mass loading of the sample catalyst and controls are determined to be 41.65 μg cat cm −2 . The Ru loading on the electrode is estimated to be 13.44, 15.21, 25.50, and 19.02 μg cm −2 for CeRuO x , SnRuO x , RuO x , and CrRuO x , respectively. The electrochemical testing is carried out in a conventional three-electrode set-up with a carbon rod and a mercurous sulfate electrode (Hg/Hg 2 SO 4 ) used as the counter electrode and reference electrode respectively. O 2 -saturated 0.5 M H 2 SO 4 was used as an electrolyte to mimic the environment of the anode in PEMWE. When conducting LSV, CA, and CP tests, the electrolyte is convected by external magnetic stirring with a speed of 300 rpm, which is sufficient to remove the visible oxygen bubble formed on the surface of the Au electrode. When collecting the CV for ECSA calculation, no magnetic stirring is applied. To conduct the CP at 100 mA cm −2 , the working electrode is prepared by air spraying the homogeneous catalyst ink on a piece of carbon paper (area 1 × 1 cm −2 ) with optimized catalyst loading (41.65 μg cat cm −2 ). All the electrochemical testing in a three-electrode set-up is conducted at 30 °C. To investigate the dissolution of M during OER, O 2 -saturated 0.1 M PBS (pH = 6) was also used as an electrolyte. For the measurement with iR -correction, R was referred to as the ohmic resistance arising from the electrolyte/contact resistance of the setup. The iR compensation was performed manually after the measurement for 100% of the R . Determine the ECSA of MRuO x The ECSAs were obtained from the electrochemical double-layer capacitance of the catalytic surface. The electrical double-layer capacitor (C DL ) were measured from double-layer charging curves using cyclic voltammograms in a non-Faradaic region with a scan rate from 5 to 25 mV s −1 . The CDL was measured by the following equation: 
    j=νC_DL
 (1) where j is the no-Faradaic capacitive current obtained from the CV curve, ν is the scan rate. The slope of j-ν curve is regarded as C DL . The ECSA is calculated from the double-layer capacitance according to: 
    ECSA=C_DL/C_S
 (2) Where C S is the specific capacitance of the sample (set as 0.035 mF cm −2 according to the previous reports). Mass activity calculation The mass activity (j mass ) of MRuO x were determined using the following equation: 
    j_mass=i_geo/m_cat×Ru wt%
 (3) where i geo is the geometric current (A) obtained from LSV, m cat is the loading of catalysts on the electrode and Ru wt% is the mass ratio of Ru in MRuO x , which is calculated from the results of ICP-OES. Calculation of the TOF The TOF of MRuO x and commercial RuO 2 were calculated based on the following equation: 
    TOF=n_O_2/n_Ru
 (4) where \({n}_{{{{{{{\mathrm{O}}}}}}}_{2}}\) is the number of oxygen per second, \({n}_{{{{{{{\mathrm{Ru}}}}}}}}\) is the number of Ru participating in the OER. Here in this work, all Ru on the electrode are assumed to be the active center during OER. Thus, the \({n}_{{Ru}}\) can be calculated as: 
    n_Ru=m_cat× Ru wt%/M_Ru
 (5) in which \({M}_{{Ru}}\) is the molar mass of Ru (101.07 g mol −1 ). \({m}_{{cat}}\) and \({Ru\; wt}\%\) are same as those in Eq. 3 . The \({n}_{{O}_{2}}\) in Eq. ( 4 ) were calculated from the LSV curve by the following equation: 
    n_O_2=i_geo/z∗ F
 (6) where \({i}_{{geo}}\) is the geometric current (A), z is the number of electrons required per oxygen molecule, F is the Faraday constant (96,484 C mol −1 ). In situ DEMS with isotope labeling In situ DEMS experiments was performed on an in situ differential electrochemical mass spectrometer provided by Linglu Instruments (Shanghai) Co. Ltd with a delay time of 1 s. A porous PTFE membrane is employed for gas-liquid separation. A typical test was carried out in a three-electrode cell with 18 O-labeled 0.5 M H 2 SO 4 or 18 O-labeled 0.1 M PBS as electrolyte and MRu 16 O x as a catalyst. Before the DEMS measurement, cyclic voltammetry was performed in the range of 0.6 − 1.2 V at 50 mV s −1 to further purge the adsorbed 16 O species on the electrode. After these processes, the in situ DEMS measurement was carried out with five consecutive LSV test on MRuO x . To exclude the influence of the abundance of 16 O in H 2 18 O, control experiments on commercial IrO 2 were carried out. The total signal intensity of O 2 is calculated to determine the OER onset potential. Electrochemical measurements in PEM electrolyzer To construct the membrane electrode assembly (MEA), SnRuO x or commercial RuO 2 were used as the anode catalysts, and commercial Pt/C (40 wt%) was used as the cathode catalyst. To prepare the anode and cathode ink, catalysts were dispersed to a mixture of isopropanol and distilled water with a ratio of 1:1. Then, Nafion® solution (5 wt%) was added in to obtain an ionomer amount of 30 wt% for an anode and 40 wt% for a cathode. After ultrasonicated for at least 1 h in a low-temperature water bath, a uniform catalyst ink can be obtained. To prepare the MEA with Nafion 212 membrane as an electrolyte, the anode and cathode catalysts were directly air sprayed on the two sides of the as-received Nafion 212 membrane in the ultrasonic spray coating system. The anode and cathode catalysts loading are controlled to be 4 mg cat cm −2 (1.46 mg Ru cm −2 ) and 1 mg cm −2 (0.4 mg Pt cm −2 ) after loading optimization. To prepare the MEA with Nafion 115 membrane as an electrolyte, the anode and cathode catalysts are first sprayed onto sheets of polytetrafluoroethylene (PTFE). After that, the PTFE-supported Pt/C, Nafion 115, and PTFE-supported anode catalysts are hot pressed together at 135 °C for 3 min under a pressure of 2 T. After cooling, the PTFE on the surface were carefully peeled off to get the catalyst-coated membrane (CCM). The anode and cathode catalysts loading are controlled to be 2 mg Ru cm −2 and 1 mg cm −2 after loading optimization. The CCM prepared was preserved in distilled water for further measurements. To construct the PEM electrolyzers for performance evaluation, the titanium felt with a thickness of 1 mm were used as the porous transport layers (PTL) in both the anode and cathode. The assembly pressure of the fixture is set to 5 N m. The active area of the electrode is measured to be 4 cm 2 . The PEM electrolyzers were operated at 80 °C with distilled water as reactant under a flow rate of 40 mL min −1 . The polarization curves were collected from 0.1 to 4.4 A cm −2 . The stability of the PEM electrolyzers were evaluated by measuring chronopotentiometry at 1 A cm −2 for 1300 h. The anode dissolution amount were monitored every 100 h by ICP-OES. DFT calculation The geometries and energies were performed by density functional theory (DFT) with Vienna ab initio simulation package (VASP) [109] , [110] , [111] , [112] , [113] , [114] , [115] , [116] . The interactions between ion cores and valence electrons were described by the projector augmented wave (PAW) method. The generalized gradient approximation with the Perdew–Burke–Ernzerhof was adopted as the exchange-correlation functional. The wave functions at each k-point were expanded with a plane wave basis set. The kinetic cutoff energy was set to 400 eV. The integration of the Brillouin zone is conducted using a 1 × 1 × 1 Monkhorst-Pack grid. The geometries were optimized using a force-based conjugate-gradient method until the energy was converged to 1.0 × 10 −4 eV/atom and the force to 0.05 eV/Å. Spin polarization was considered in our current study and the U parameter used for M atoms was 4.0 eV. The structure of M 0.5 Ru 0.5 O 2 were based on the results from XRD refinement. M 0.5 Ru 0.5 O 2 (110) was constructed by cutting the bulk M 0.5 Ru 0.5 O 2 alone in 110 direction and four layers were selected. For defective structures, Ru and M vacancies are considered (see Supplementary Note 4 ). During the optimization, the up-layer atoms were allowed to relax and the atoms in the last layer were fixed to keep the bulk structure. A vacuum layer of 15 Å was used along the c direction normal to the surface to avoid periodic interactions. To illustrate the activity of AEM (adsorbate evolution mechanism) and LOM (a lattice-oxygen-mediate mechanism), the free energy diagrams was estimated as follows: 
    ΔG=ΔE+ΔZPE-TΔS
 where ΔE is the total energy change based on the DFT calculations, ZPE and S is the zero-point energy and entropy, respectively, T is the temperature (here, 298.15 K is selected). The free energy of (H + + e - ) at standard conditions is assumed as the energy of 1/2 H 2 .